MCIDASmutations result in a mucociliary clearance disorder with reduced generation of multiple motile cilia Reduced generation of multiple motile cilia (RGMC) is a rare mucociliary clearance disorder. Affected persons suffer from recurrent infections of upper and lower airways because of highly reduced numbers of multiple motile respiratory cilia. Here we report recessive loss-of-function and missense mutations in MCIDAS -encoding Multicilin, which was shown to promote the early steps of multiciliated cell differentiation in Xenopus . MCIDAS mutant respiratory epithelial cells carry only one or two cilia per cell, which lack ciliary motility-related proteins (DNAH5; CCDC39) as seen in primary ciliary dyskinesia. Consistent with this finding, FOXJ1-regulating axonemal motor protein expression is absent in respiratory cells of MCIDAS mutant individuals. CCNO , when mutated known to cause RGMC, is also absent in MCIDAS mutant respiratory cells, consistent with its downstream activity. Thus, our findings identify Multicilin as a key regulator of CCNO/FOXJ1 for human multiciliated cell differentiation, and highlight the 5q11 region containing CCNO and MCIDAS as a locus underlying RGMC. Each ciliated respiratory cell is covered by multiple cilia, beating vigorously in a coordinated beating pattern to move inhaled particles, cell detritus and microbes trapped in the mucus towards the throat [1] , [2] . This mechanism referred to as mucociliary clearance is important to prevent chronic airway disease. Congenital disorders impairing mucociliary clearance such as primary ciliary dyskinesia (PCD; MIM244400) and cystic fibrosis (MIM219700) are well-known causes of recurrent upper and lower respiratory tract infections. Whereas in PCD and cystic fibrosis either dysfunction of cilia beating or abnormal mucus viscosity causes defective mucociliary clearance, we recently identified a distinct mucociliary clearance disorder characterized by reduced generation of multiple motile cilia (RGMC) because of mutations in CCNO -encoding Cyclin O (ref. 3 ). Cyclin O is required to generate the basal bodies necessary for multiple cilia formation by promoting a process of centriole assembly and maturation that is likely unique to these cells. Strikingly, CCNO lies adjacent to genes on chromosome 5q11 that have also been implicated in early aspects of multiciliated cell differentiation [4] , [5] , [6] . One of these, MCIDAS , encodes a nuclear protein, referred to as Multicilin, which promotes multiciliated cell formation in Xenopus skin and kidney tissue as well as in mouse airway epithelium cell cultures [3] , most likely as a transcriptional co-activator. Here we show that mutations in MCIDAS cause RGMC in humans, emphasizing the importance of the chromosomal region 5q11 as a key locus for multiciliated cell differentiation. 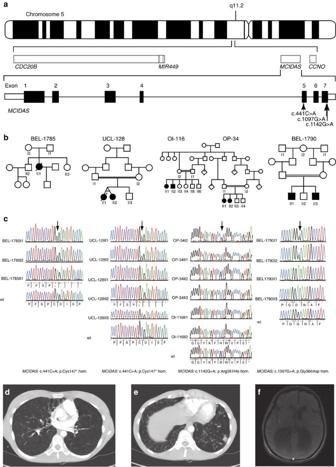Figure 1:MCIDASmutations cause chronic destructive airway disease. (a) Schematic overview of chromosome 5, harbouring the genomic region ofCCNO, MCIDAS, CDC20BandMiR449. Overview ofMCIDAS; all mutations are marked with arrows. (b) Pedigrees of the families BEL-1785, UCL-128, OI-116/OP-34 and BEL-1790 with recessiveMCIDASmutations. (c) DNA sequence reads of the affected families compared with wild-type sequence. The mutations are marked with an arrow. (d,e) The computed tomography (CT) scans of BEL-1785 showsitus solitus, chronic airways disease with bronchiectasis and mucus plugging. (f) Magnetic resonance imaging of the brain of UCL-128 II1 shows enlarged brain ventricles (hydrocephalus). Mutational analysis identifies recessive mutations in MCIDAS Whole-exome sequencing in the Belgian individual BEL-1785II1, previously reported as a patient with ciliary aplasia [7] , revealed a homozygous nonsense mutation c.441C>A in exon 5 of MCIDAS ( Supplementary Table 1 ). This mutation results in a premature stop codon (p.Cys147*), predicting a truncated protein before the coiled-coil domain (CCDC) of the protein, which is essential for its function. The mutation was confirmed by Sanger sequencing and heterozygous carrier status was demonstrated in both parents, consistent with autosomal recessive inheritance ( Fig. 1c ). MCIDAS (CCDS54853) located on chromosome 5q11, consists of seven exons encoding a 1,736-bp transcript and 385 amino-acid protein. We next performed Sanger DNA sequencing of all coding exons of MCIDAS , including the exon–intron boundaries, in 59 families with absence of CCNO mutations. All affected individuals had reduced numbers of cilia demonstrated by transmission electron microscopy (TEM), immunofluorescence (IF) staining or both. Sequence analyses revealed biallelic mutations in three additional families with a total of eight individuals. In the two affected patients of the UCL-128 Pakistani family, the same c.441C>A (p.Cys147*) was detected ( Fig. 1c ). In one large Israeli consanguineous pedigree OI-116/OP-34, which had previously been reported by Soferman et al. [8] , a homozygous missense mutation in a highly conserved region was identified (c.1142 G>A; p.Arg381His) in four affected members ( Fig. 1b,c ). A homozygous mutation (c.1097 G>A; p.Gly366Asp) was found in two brothers from the consanguineous Turkish family BEL-1790. All mutations were not present in the 1,000 genomes database and segregated consistently with autosomal-recessive inheritance. Figure 1: MCIDAS mutations cause chronic destructive airway disease. ( a ) Schematic overview of chromosome 5, harbouring the genomic region of CCNO, MCIDAS, CDC20B and MiR449 . Overview of MCIDAS ; all mutations are marked with arrows. ( b ) Pedigrees of the families BEL-1785, UCL-128, OI-116/OP-34 and BEL-1790 with recessive MCIDAS mutations. ( c ) DNA sequence reads of the affected families compared with wild-type sequence. The mutations are marked with an arrow. ( d , e ) The computed tomography (CT) scans of BEL-1785 show situs solitus , chronic airways disease with bronchiectasis and mucus plugging. ( f ) Magnetic resonance imaging of the brain of UCL-128 II1 shows enlarged brain ventricles ( hydrocephalus ). Full size image Clinical phenotype of affected individuals The individuals with biallelic MCIDAS mutations displayed typical signs of a mucociliary clearance disorder with chronic recurrent infections of the upper (rhinitis, otitis media, nasal polyps and sinusitis) and lower airways (recurrent pneumonia, bronchiectasis, chronic obstructive airway disease; Fig. 1d,e ). Postnatal respiratory distress syndrome was present in all individuals. Two individuals died because of respiratory insufficiency: BEL-1785 at the age of 27 years; UCL-128II1 at the age of 19 years, two years after lung transplantation. BEL-1790II1 was chronically oxygen dependent at the age of 27 years. 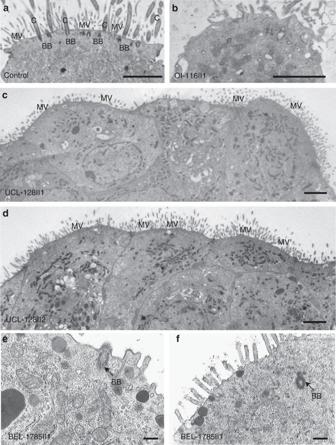Figure 2: Transmission electron microscopy (TEM) demonstrates severe reduction of cilia and basal bodies. (a) Respiratory epithelial cells from a healthy control individual showing basal bodies (BB) on the apical membrane nucleating multiple motile cilia (C) and microvilli (MV) at the apical region. (b–f) Respiratory epithelial cells of affected individuals (OI-116 II1, UCL-128 II1, UCL-128 II2, BEL-1785 II1). Scale bars, 2 μm. Nasal nitric oxide measurements were low in the individuals BEL-1785, UCL-128II1, UCL-128II2; OI-116II1, OI-116II2 and BEL-1790II1 and BEL-1790II3 ( Supplementary Table 2 ) resembling diagnostic findings encountered in PCD individuals. All nine individuals with biallelic MCIDAS mutations had normal situs composition, which is consistent with previous reports indicating no functional role of Multicilin for left–right determination during early embryogenesis [4] . BEL-1785 became pregnant only after in vitro fertilization. The two affected UCL-128 twins, as well as the two brothers BEL-1790II1 and BEL-1790II3 and BEL-1785, had arrested hydrocephalus ( Fig. 1f ). Possibly, the clinical manifestations of female infertility (BEL-1785) and hydrocephalus (UCL-128; BEL-1790; BEL-1785) are related to RGMC of multiciliated fallopian tube and multiciliated ependymal cells, respectively, both densely populated with motile cilia. Ependymal ciliary motility has been implicated to have an important role in the prevention of hydrocephalus in human and mice [9] . In addition, defective motility of fallopian tube cilia has been suspected possibly related to female infertility [10] . p.Gly366Asp/p.Arg381His disable endogenous mcidas-activity To verify the effect of the detected amino-acid exchanges c.1142 G>A; p.Arg381His in the family OI-116/OP-34 and c.1097 G>A; p.Gly355Asp in the family BEL-1790, an equivalent mutation was introduced in the Xenopus mcidas (Arg370His/Gly355Asp) by PCR and tested in a gain-of-function experiment. As shown previously, ectopic expression of wild-type mcidas in Xenopus embryos readily induced the formation of ectopic multiciliated cells. However, ectopic expression of mcidas p.Arg370His and p.Gly355Asp in embryos did not induce ectopic multiciliated cells, but instead led to a reduction in cell number and an increase in cell size, a phenotype known from embryos expressing a form of mcidas lacking the conserved C-terminal TIRT domain, mcidas Δ334-374 (ref. 4 ). The fact that mcidas p.Arg370His and p.Gly355Asp show a similar phenotype, as mcidas Δ334–374 indicates that these mutations disable the activity of endogenous mcidas in multiciliated cell differentiation ( Supplementary Fig. 1 ). Expression of MCIDAS, CCNO and CDC20B MCIDAS, CCNO and miRNA449a-c within CDC20B lie adjacent to each other in a conserved genomic region. We next examined how the expression of these genes varies at different time points during the ciliogenesis procedure on cultured human nasal epithelial cells using quantitative PCR. The expression of these three genes was very low during the monolayer phase, at a time point when there is only de-differentiation and no stimulation of the formation of multiciliated cells [11] . Shortly after the cells were brought into the suspension culture to induce ciliogenesis and the formation of multiciliated cells, the expression of the three genes increased equally ( Supplementary Fig. 2 ). Thus, the coordinate expression of MCIDAS , CCNO and CDC20B is a conserved feature of multiple motile cilia (MMC) generation and further implicates MCIDAS in this process. TEM shows reduced cilia number and basal body mislocalization Consistent with defective generation of MMC, we found either complete absence or severely reduced numbers of cilia in BEL-1785, UCL-128II1/II2, OI-116II1/II2 and BEL-1790II1/II3 by TEM of respiratory epithelial cells ( Fig. 2 ). The apical cell regions showed normal microvilli composition but severe decrease of basal bodies (specialized centrioles that nucleate ciliary axonemes) indicating that MCIDAS dysfunction results in a marked reduction of centrioles, which are essential for MMC generation. Occasionally, we found basal bodies mislocalized in the cytoplasm. Similar TEM results had been reported previously for OI-116II1/II2, OP-34II1/II2 and BEL-1785 7+8 . To corroborate our findings, we performed in vitro ciliogenesis experiments of primary respiratory cells in BEL-1785, UCL-128II1/II2 and BEL-1790II1/II3 and confirmed the defect in MMC generation. Our TEM results resembled findings reported in CCNO mutant respiratory cells [3] . Figure 2: Transmission electron microscopy (TEM) demonstrates severe reduction of cilia and basal bodies. ( a ) Respiratory epithelial cells from a healthy control individual showing basal bodies (BB) on the apical membrane nucleating multiple motile cilia (C) and microvilli (MV) at the apical region. ( b – f ) Respiratory epithelial cells of affected individuals (OI-116 II1, UCL-128 II1, UCL-128 II2, BEL-1785 II1). Scale bars, 2 μm. Full size image To further investigate the observed MMC generation defect, nasal respiratory epithelial cells were obtained for IF microscopy from the affected individuals OI-116II1/II2, BEL-1790II1/II3 and healthy controls. Staining with antibodies targeting acetylated α-tubulin showed a severe reduction of MMCs, compared with healthy controls, respectively. Quantification of cilia revealed that most respiratory cells were completely devoid of any cilia. The few respiratory cells with cilia had only one or two cilia per ciliated cell. Thus, our findings confirm a severe defect of MMC generation in MCIDAS mutant cells resembling findings present in CCNO mutant cells [3] . To further characterize Multicilin function, we analysed protein expression in control respiratory cells by western blot and IF analysis. Multicilin localized to the nucleus in control cells destined for multiciliated cell differentiation, whereas its expression is absent or very weak in fully differentiated ciliated respiratory cells ( Fig. 3a ). In contrast, Multicilin was absent or severely reduced in the samples of the affected individuals OI-116II1 and OI-116II2, respectively ( Fig. 3b ). 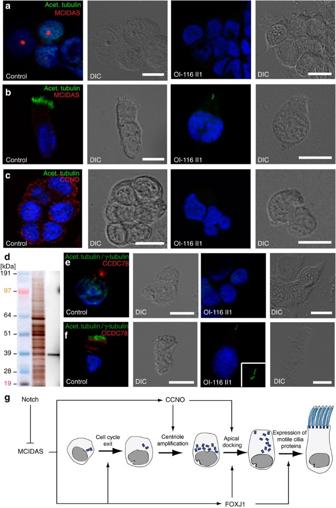Figure 3: The nuclear factor MCIDAS acts upstream of CCNO in the acentriolar deuterosome-mediated pathway. Respiratory epithelial cells from healthy control individuals (a,bleft panels) and affected individual OI-116 II1 (a,bright panels) were stained with antibodies directed against MCIDAS and acetylated α-tubulin. MCIDAS is strongly expressed in the nucleus (red) of undifferentiated respiratory cells destined for multiciliated cell differentiation (a; left panels), whereas nuclear expression is very weak or absent in fully differentiated multiciliated cells (bleft panels). InMCIDASmutant cells, MCIDAS was not detectable in undifferentiated or differentiated respiratory cells (a,bright panels). (c) CCNO was absent in respiratory cells of OI-116 II1 (right panels) compared with control (red; left panels), which is consistent with CCNO acting downstream of MCIDAS. (d) Anti-MCIDAS detects a protein of the expected size (38 kDa) in respiratory cell lysates by western blot analysis. (e,fleft panels) CCDC78, a protein known to be involved in the deuterosome-dependent centriole assembly, is present in control respiratory cells in the apical cytoplasm (centriole amplification) and in the vicinity of basal bodies (fully differentiated ciliated cells). In contrast, inMCIDASmutant cells, expression ofCCDC78(e,fright panels) is not detectable in respiratory cells of any stage of multiciliated cell differentiation, which is consistent with MCIDAS functioning in the deuterosome-mediated pathway of centriole assembly. (g) Schematic depicting the dual role of MCIDAS in the differentiation of multiciliated cells and the generation of multiple motile cilia. NOTCH functions as a repressor of MCIDAS. FOXJ1 and CCNO act downstream of MCIDAS. Nuclei are stained with Hoechst33342; scale bar, 10 μm. Figure 3: The nuclear factor MCIDAS acts upstream of CCNO in the acentriolar deuterosome-mediated pathway. Respiratory epithelial cells from healthy control individuals ( a,b left panels) and affected individual OI-116 II1 ( a , b right panels) were stained with antibodies directed against MCIDAS and acetylated α-tubulin. MCIDAS is strongly expressed in the nucleus (red) of undifferentiated respiratory cells destined for multiciliated cell differentiation ( a ; left panels), whereas nuclear expression is very weak or absent in fully differentiated multiciliated cells ( b left panels). In MCIDAS mutant cells, MCIDAS was not detectable in undifferentiated or differentiated respiratory cells ( a , b right panels). ( c ) CCNO was absent in respiratory cells of OI-116 II1 (right panels) compared with control (red; left panels), which is consistent with CCNO acting downstream of MCIDAS. ( d ) Anti-MCIDAS detects a protein of the expected size (38 kDa) in respiratory cell lysates by western blot analysis. ( e,f left panels) CCDC78, a protein known to be involved in the deuterosome-dependent centriole assembly, is present in control respiratory cells in the apical cytoplasm (centriole amplification) and in the vicinity of basal bodies (fully differentiated ciliated cells). In contrast, in MCIDAS mutant cells, expression of CCDC78 ( e , f right panels) is not detectable in respiratory cells of any stage of multiciliated cell differentiation, which is consistent with MCIDAS functioning in the deuterosome-mediated pathway of centriole assembly. ( g ) Schematic depicting the dual role of MCIDAS in the differentiation of multiciliated cells and the generation of multiple motile cilia. NOTCH functions as a repressor of MCIDAS. FOXJ1 and CCNO act downstream of MCIDAS. Nuclei are stained with Hoechst33342; scale bar, 10 μm. Full size image Multicilin regulates CCNO and FOXJ1 expression Previously, we reported that CCNO acts downstream of MCIDAS [3] and that CCNO deficiency results in reduced MMC generation. To corroborate these findings, we analysed CCNO expression in MCIDAS mutant respiratory cells. Consistent with up-stream function of MCIDAS, we found that analysed CCNO expression was severely reduced or absent in mutant cells ( Fig. 3c ), providing more evidence that both Multicilin and CCNO function in the same pathway and defects of either protein cause inherited RGMC defects. Western blot analysis identified a specific band of the expected size in respiratory cell lysates ( Fig. 3d ). Multicilin has previously been shown to induce expression of multiciliogenesis-related genes, such as CCNO , required for centriole assembly and docking in multiciliated cells and FOXJ1 , necessary for centriole docking and transcription control of ciliary motility-related proteins [3] , [12] . To further examine how Multicilin promotes multiciliogenesis, we analysed whether the few residual cilia present at the cell surface contain axonemal motor proteins such as the outer dynein arm heavy chain DNAH5 and the nexin-dynein regulatory complex-related protein CCDC39. Interestingly, in contrast to CCNO mutant cells, MCIDAS mutant cells lacked any axonemal motility-related proteins ( Fig. 4a,b ). This indicates that in MCIDAS mutant cells not only the number of MMCs is severely reduced, but also the expression of ciliary motility-related proteins (for example, DNAH5; CCDC39) is disrupted. We therefore stained FOXJ1 (transcriptional control of ciliary motility-related proteins) in respiratory epithelial cells of affected and healthy controls ( Fig. 4f ). Consistent with absent axonemal motility-related proteins (DNAH5; CCDC39), FOXJ1 was also absent from the nuclei in MCIDAS mutants. Thus, our findings in human respiratory cells fit with previously reported results indicating that Multicilin regulates CCNO (MMC generation) and FOXJ1 (motile cilium) generation [4] . 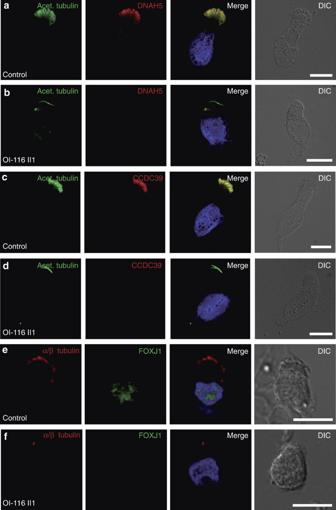Figure 4: The number of cilia is markedly reduced and residual cilia lack axonemal motor proteins. (a–d) Respiratory epithelial cells from control (a,c) and OI-116 II1 (b,d) with recessiveMCIDASmutations were labelled with antibodies against axonemal motor protein outer dynein arm heavy chain DNAH5 (red;a,b) and the dynein regulator complex-related protein CCDC39 (red;c,d), respectively. Cilia were marked with acetylated α-tubulin as axonemal control (green;a–d). (e,f) FOXJ1 localizes to the nucleus in healthy control cells (e, green) and is absent in affected individuals (f) consistent with FOXJ1 acting downstream of MCIDAS. Cilia were stained for α/β-tubulin as axonemal control (red;e,f). Nuclei stained with Hoechst33342; scale bar, 10 μm. Figure 4: The number of cilia is markedly reduced and residual cilia lack axonemal motor proteins. ( a – d ) Respiratory epithelial cells from control ( a , c ) and OI-116 II1 ( b , d ) with recessive MCIDAS mutations were labelled with antibodies against axonemal motor protein outer dynein arm heavy chain DNAH5 (red; a , b ) and the dynein regulator complex-related protein CCDC39 (red; c , d ), respectively. Cilia were marked with acetylated α-tubulin as axonemal control (green; a – d ). ( e , f ) FOXJ1 localizes to the nucleus in healthy control cells ( e , green) and is absent in affected individuals ( f ) consistent with FOXJ1 acting downstream of MCIDAS. Cilia were stained for α/β-tubulin as axonemal control (red; e , f ). Nuclei stained with Hoechst33342; scale bar, 10 μm. Full size image MCIDAS is required for the deuterosome-mediated acentriolar pathway The massive expansion of mother centrioles that underlies multiciliated cell differentiation occurs on novel structures, called deuterosomes, which can be induced ectopically by Multicilin [4] . Recently, two proteins required for deuterosome formation have been identified, DEUP1 and CCDC78 (refs 13 , 14 ). We therefore explored whether the deuterosome pathway is still active in MCIDAS mutant cells, by analysing the expression of CCDC78 in respiratory epithelial cells from MCIDAS mutant individuals. These cells failed to express CCDC78 , providing genetic evidence that MCIDAS is required the deuterosome-mediated, acentriolar assembly pathway in human respiratory cells ( Fig. 3e,f ). In conclusion, we found mutations in MCIDAS in nine individuals from four families with a congenital mucociliary clearance disorder with RGMC. MCIDAS has previously been shown to induce generation of multiciliated cells in Xenopus skin and kidney tissue as well as in mouse airway epithelium cell cultures. We have now shown that MCIDAS is also essential for generation of multiciliated cells in human respiratory epithelium and that its expression is upregulated during a critical period of cilia generation. Mutations in CCNO result in a RGMC disorder with some residual ciliary motility (type CCNO) and CCNO mutant cilia do not exhibit obvious axonemal structural or beating defects, which is distinct from PCD that is defined by congenital defects of respiratory cilia beating. However, mutations in MCIDAS cause a RGMC disorder with few cilia that are immotile. This defect can be also categorized as a novel PCD variant, because MCIDAS mutant cilia display severe axonemal defects (lack of ciliary motility-related proteins) and are immotile, and therefore meet the definition criteria of PCD. Our genetic findings highlight the importance of the genomic region containing CCNO and MCIDAS as a key locus for multiciliated cell differentiation ( Fig. 3g ) and will aid early diagnosis of this chronic respiratory disorder. Patients We obtained signed and informed consent from affected individuals using protocols approved by the Institutional Ethics Review Board of the University of Münster, Freiburg and collaborating institutions. To maintain privacy protection of the affected individual (BEL-1785), data of the whole-exome analysis were not deposited in either a public or controlled-access database. Exome sequencing A DNA library of the index case (BEL-1785) was prepared with DNA library preparation kit TruSeq DNA Sample Prep kit v2 (Illumina) according to the manufacturer’s recommendations. A partial exome was captured from this DNA library by the Exome capturing kit SeqCap EZ Human Exome Library v3.0 (Nimblegen) according to the manufacturer’s recommendations. For sequencing, the TruSeq PE Cluster Kit v3-cBot-HS and TruSeq SBS Kit v3-HS kits (Illumina) were used according to the standard protocols of the manufacturer. Sequencing was performed on a HiSeq 2000 sequencing apparatus (Illumina). The reads were aligned to the hg19 reference sequence ( http://hgdownload.soe.ucsc.edu/goldenPath/hg19/database ) using CLC Genomics Workbench software CLCbio ( http://www.clcbio.com/ ). Variants were called using the Probabilistic Variant Detection algorithm in CLC Genomics Workbench. This algorithm is a combination of a Bayesian model and a Maximum Likelihood approach to calculate prior and error probabilities for the Bayesian model. The significance for variant probability (the posterior probability from the Bayesian approach) was set to at least 95. Using CLC Genomics Workbench, only variants at positions were called for which the read depth was at least 10 reads and that were located in the coding region and flanking 30 nucleotides of the RefSeq genes ( http://genome.ucsc.edu/ ), and that were not found in the SNP137 ( http://hgdownload.soe.ucsc.edu/goldenPath/hg19/database/ ) database, nor in in-house whole-exome variants found in 12 characterized PCD patients. Mutation analysis Standard methods were used to isolate Genomic DNA directly from blood or lymphocyte cultures after Ebstein–Barr virus-mediated transformation. Six genomic fragments comprising all exons of MCIDAS were amplified as described before [15] . IF analysis Respiratory epithelial cells were obtained by nasal brush biopsy (Engelbrecht Medicine and Laboratory technology) and suspended in cell culture medium. Samples were spread onto glass slides, air dried and stored at −80 °C until use. Spheroid cultures from nasal brushings were performed as reported [16] . Before incubation with the primary antibody (2–3 h at room temperature or overnight at 4 °C) and secondary antibody (25 min room temperature), cells were treated with 4% paraformaldehyde or 100% ice-cold methanol, 0.2% Triton X-100 and 1% skim milk. Rabbit polyclonal antibody directed against DNAH5 was previously reported [17] . Rabbit polyclonal anti-CCNO (1:50), anti-MCIDAS (alias RP11-528L24.3, 1:500), anti-CCDC39 (1:300), anti-CCDC78 (1:100) were obtained from Atlas Antibodies. Mouse monoclonal antibody directed against acetylated tubulin (1:10,000) and γ-tubulin (1:500) were obtained from Sigma and mouse monoclonal anti-FOXJ1 (1:200) from eBiosciences. Rabbit polyclonal anti-CEP164 (1:200) was purchased from Acris Antibodies and rabbit polyclonal anti-α/β-tubulin (1:300) from Cell Signaling. Highly cross absorbed secondary antibodies, including Alexa Fluor 488-conjugated goat antibodies to mouse (1:1,000, A11029) and Alexa Fluor 546-conjugated goat antibodies to rabbit (1:1,000, A11035) were from Molecular Probes (Invitrogen). DNA was stained with Hoechst33342 (1:1,000, 14533-100MG, Sigma). IF images were taken with a Zeiss Apotome Axiovert 200 and processed with AxioVision 4.8 and Adobe CS4. Immunoblotting Protein extracts were prepared from human respiratory epithelial cell cultures as described previously [15] . Proteins were separated on a NuPAGE 4–12% bis-tris gel (Invitrogen) and blotted onto a polyvinylidene difluoride membrane (GE Healthcare). Polyvinylidene difluoride filtres were washed three times in TBST (10 min each) before blocking in 5% skim milk in TBST overnight at 4 °C. Filtres were incubated with primary antibody (diluted in 5% skim milk in TBST) for 3 h at room temperature or overnight at 4 °C. Filtres were washed three times (10 min each) and then incubated with secondary antibody goat anti-rabbit HRP antibody (1:3,000; NA934, GE Healthcare) for 1 h at room temperature. Filtres were then washed four times and developed by ECL using Prime Western Blotting Detection Reagent (GE Healthcare). Images were digitally acquired using a FUSION-SL Advance Imager (PeqLab) and modified for contrast using Adobe Photoshop v. CS4 (Adobe). TEM Nasal biopsies were taken from the middle turbinate. The sample was fixed in 2.5% glutaraldehyde and washed with 1.3% Osmiumacid. The samples were embedded in 1,2-Epoxypropan-Epon-mixture (1:1) overnight at 4 °C. After polymerization, several sections were picked out onto copper grids. The sections were stained with Reynold’s lead citrate. Transmission electron microscopy was performed with the Philips CM10 (Philips). Ciliogenesis procedure Respiratory epithelial cells were obtained by punch biopsy and brought into a sequential monolayer-suspension culture. Part of the biopsy specimen was prepared for TEM. TEM was again performed after ciliogenesis, to exclude secondary damage. First, the biopsy sample was brought into a monolayer culture (on collagen layer), to induce de-differentiation of the respiratory epithelium and loss of cilia. The dissociated nasal epithelial cells were seeded and cultured in several T25 culture flasks coated with a collagen coat (medium DMEM-Ham's F12 from Life Technologies, supplemented with AB (50 U ml −1 penicillin and 50 μg ml −1 streptomycin) and 2% Ultroser G (Life Technologies). After 3 weeks, when all the cells had become cuboidal and lost their cilia, the cells were brought into a suspension culture medium DMEM-Ham's F12 from Life Technologies supplemented with AB (50 U ml −1 penicillin and 50 μg ml −1 streptomycin) and 10% NU-Serum (Becton Dickinson), to induce spheroid formation and differentiation in a ciliated epithelium. In this way, de novo ciliogenesis was induced and secondary defects could be reliably excluded. Real-time PCR For real-time PCR (quantitative PCR), human nasal epithelial cells were isolated from surgical material from three control patients (suffering from nasal polyps) and brought into a monolayer-suspension culture, showing normal ciliary activity. Cells were collected at different time points during ciliogenesis (1 week monolayer, 2 weeks monolayer, 3 weeks monolayer, 3 days suspension, 1 week suspension, 10 days suspension, 2 weeks suspension and 3 weeks suspension). The collected cells were stored at −80 °C. After 6 weeks of culture, RNA was extracted from the cultured ciliated epithelial cells using the RNeasy Mini Kit (Qiagen). Quantitative PCR was performed on three neighbouring genes: MCIDAS, CCNO and CDC20B . RNA (1 μg) extracted from cultured epithelial cells of the three control patients at different time points during ciliogenesis was reversed transcribed into cDNA using Superscript reverse transcriptase II (Invitrogen). The real-time PCR (quantitative PCR) reaction was performed for each patient on the three genes in 96-well clear optical reaction plates (Applied Biosystems). Each reaction was performed in 25 μl solutions containing 2 μl of cDNA, × 1 SYBR Green PCR Master Mix (Applied Biosystems) and 200 nM of each sense and antisense primer. The reaction conditions were set at 95 °C for 10 min, followed by 40 cycles of 95 °C for 15 s and 60 °C for 1 min and run on the ABI 7500 system (Applied Biosystems). To correct for the total amount of cDNA present in the sample, two different housekeeping genes β2M (beta 2-microglobulin) and PPIA (Cyclophilin A) were amplified in the same assay. Supplementary Fig. 2 shows the negative Ct (threshold cycle) value for the three genes in comparison with the geometric average of the two endogenous housekeeping genes. Expression analysis of MCIDAS, CCNO and CDC20B RNA was reversed transcribed into cDNA using superscript reverse transcriptase II (Invitrogen). Forward and reverse primers were chosen in two different exons. Amplification was performed using AmpliTaq Gold DNA polymerase kit (Roche) and primers were used at 10 pmol of each primer (forward and reverse). Amplification was performed using the following temperature profile: 5 min at 95 °C; 35 cycles composed 30 s at 95 °C, 30 s at 56 °C and 1 min at 72 °C; 5 min at 72 °C and 4 °C. Primers used for PCR are listed in Supplementary Table 3. How to cite this article: Boon, M. et al. MCIDAS mutations result in a mucociliary clearance disorder with reduced generation of multiple motile cilia. Nat. Commun. 5:4418 doi: 10.1038/ncomms5418 (2014).